Three-fold rotational defects in two-dimensional transition metal dichalcogenides As defects frequently govern the properties of crystalline solids, the precise microscopic knowledge of defect atomic structure is of fundamental importance. We report a new class of point defects in single-layer transition metal dichalcogenides that can be created through 60° rotations of metal–chalcogen bonds in the trigonal prismatic lattice, with the simplest among them being a three-fold symmetric trefoil-like defect. The defects, which are inherently related to the crystal symmetry of transition metal dichalcogenides, can expand through sequential bond rotations, as evident from in situ scanning transmission electron microscopy experiments, and eventually form larger linear defects consisting of aligned 8–5–5–8 membered rings. First-principles calculations provide insights into the evolution of rotational defects and show that they give rise to p-type doping and local magnetic moments, but weakly affect mechanical characteristics of transition metal dichalcogenides. Thus, controllable introduction of rotational defects can be used to engineer the properties of these materials. Point and line defects strongly influence electronic, optical, thermal and mechanical properties of solids, either with overall detrimental (for example, defect-induced embrittlement of reactor steels) or beneficial (doping of semiconductors) effect on the materials characteristics, calling on careful investigations of their atomic structure. Aberration-corrected transmission electron microscopy (TEM) made it possible to study the structure and behaviour of defects on atomic scale in real time, and has provided many insights into defect dynamics. In sp 2 -hybridized hexagonal carbon systems, for example, carbon nanotubes [1] or graphene [2] , [3] , Stone–Wales transformations [4] representing rotations of C–C bonds by 90° ( Fig. 1a,b ) have been observed. Such transformations can be regarded as an elementary step that not only gives rise to topological defects [5] , [6] , but are also responsible for plastic deformation [7] , [8] , rippling [9] and grain boundary motion [10] . 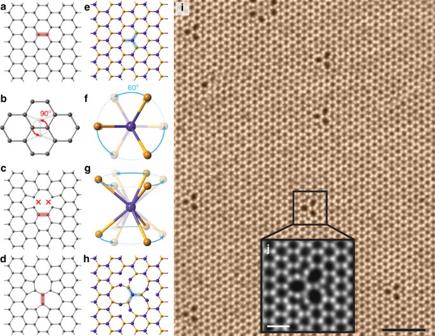Figure 1: Model of rotational defect in graphene and TMDs. (a) Atomic model of graphene. (b) Top view of the Stone–Wales transformation, showing 90° rotation of a carbon bond. (c) Atomic model of graphene with a divacancy. (d) The atomic model of SW-transformed graphene divacancy. (e) Atomic model of TMDs with a structural formula MX2, the top view. The orange spheres represent chalcogen atoms, the blue ones the metal atoms. (f,g) Triple M–X bonds showing 60° rotation from the top and perspective views. (h) The atomic model of trefoil defect. Three M–X bond pairs marked by blue bars are 60° rotated from those ine. (i) A typical ADF image of WSe2observed at 500 °C. The density of trefoil defect is found to be about 5.1%. Scale bar, 2 nm. (j) The magnified ADF image from the black square ini. Scale bar, 0.5 nm. Figure 1: Model of rotational defect in graphene and TMDs. ( a ) Atomic model of graphene. ( b ) Top view of the Stone–Wales transformation, showing 90° rotation of a carbon bond. ( c ) Atomic model of graphene with a divacancy. ( d ) The atomic model of SW-transformed graphene divacancy. ( e ) Atomic model of TMDs with a structural formula MX 2 , the top view. The orange spheres represent chalcogen atoms, the blue ones the metal atoms. ( f , g ) Triple M–X bonds showing 60° rotation from the top and perspective views. ( h ) The atomic model of trefoil defect. Three M–X bond pairs marked by blue bars are 60° rotated from those in e . ( i ) A typical ADF image of WSe 2 observed at 500 °C. The density of trefoil defect is found to be about 5.1%. Scale bar, 2 nm. ( j ) The magnified ADF image from the black square in i . Scale bar, 0.5 nm. Full size image In two-dimensional (2D) materials with trigonal symmetry, for example, h-BN [11] , [12] , [13] , [14] or transition metal dichalcogenides (TMDs) [15] , [16] , [17] , [18] , [19] , [20] , point and line defects have been observed, but Stone–Wales rotational defects are not expected due to the polar nature of chemical bonds in such systems. On the other hand, a 60° rotation of three bonds centred on a metal atom, as schematically shown in Fig. 1e–g , would preserve the heteroatomic nature of bonding and the trigonal lattice symmetry, resulting in the formation a ‘trefoil’-shaped defect ( Fig. 1h ). This gives rise to the fundamental question: can such transformations occur in stoichiometric or atom-deficient 2D systems with trigonal symmetry, and if yes, what kind of defects they would produce and how would these defects affect the properties of the material. In the following, we present observations of such rotational defects. By combing scanning TEM (STEM) experiments with first-principles calculations, we show that such rotational defects exist in chalcogen-deficient TMDs and that the trefoil defect ( Fig. 1j ) is the simplest example in a series of bond rotation-mediated transformations in the TMDs. By sequential rotations of metal–chalcogen (M–X) bonds, the rotational defects can expand in size and also migrate in the lattice, or form one-dimensional domain boundaries. The formation and evolution of the defects are mediated by chalcogen vacancies induced by the electron-beam irradiation. Atomic structure of rotational defects in TMDs Figure 1i presents examples of trefoil defects in WSe 2 , which were found abundant at elevated temperatures. A comparison of the experimental STEM images with the simulated ones based on possible atomic structures ( Supplementary Fig. 2 ) indicated that the system is Se deficient due to electron-beam irradiation. Similar trefoil-shaped defects also exist in graphene as reconstructed divacancies, but there the C–C bond is rotated by 90° as shown in Fig. 1c,d . 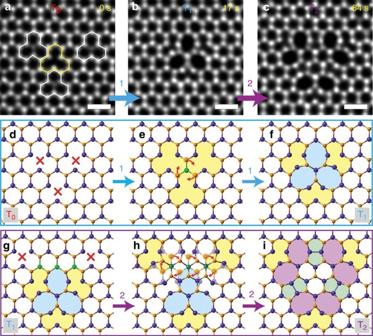Figure 2: Structure, formation and evolution of rotational defect in WSe2. The filtered ADF images of WSe2of (a) SVSe(white polygon) and DVSe(yellow polygon), (b) T1defect and (c) T2defect. (d–f) The atomic model of T0to T1transformation including the creation of three DVSe(red crosses) (d) and a 60° rotation of three pairs of W–Se bonds around the W atom (green)eto form T1with three octagons (blue;f). (g–i) The atomic model of T1to T2transformation. (g) Two DVSeare created at the vicinity of T1defect. (h) Seven pairs of W–Se bond rotations according to the W atoms marked by green color. (i) The T2defect. Scale bar, 0.5 nm. Figure 2a–c shows the filtered annular dark-field (ADF) images of three different Se-deficient WSe 2 structures. In Fig. 2a , one can see two distinct image contrasts of the vacancies at the Se sites, corresponding to single Se vacancies (SV Se , white polygon) and double vacancies (DV Se , yellow polygon), respectively. At t =17 s, a new WSe 2 defect of three-fold rotational symmetry, consisting of three eight-membered rings, resembling a trifoliate leaf, suddenly appears ( Fig. 2b ). We designate this three-fold symmetrical trefoil defect as the ‘first-order rotational defect’ or ‘T 1 ’ (with the lattice keeping the original symmetry being ‘T 0 ’). A model of the defect transformation from T 0 to T 1 is presented in Fig. 2d–f . The trefoil defects were always observed in W-centred configuration, but never in the equally possible Se-centred configuration, indicating the crucial role of the Se vacancies in the formation of the defect. We stress that the actual transformation mechanism may include not only bond rotations, but also the migration and rearrangements of Se atoms in the region with high vacancy concentration. By quantitative STEM simulations, the metal-centred T 1 defect with 3DV included (T 1 (3DV)) is a best fit to the experimental results ( Supplementary Figs 1 and 2 and Supplementary Note 1 ). We have also observed such defects in WS 2 and MoSe 2 , but not in MoS 2 . Figure 2: Structure, formation and evolution of rotational defect in WSe 2 . The filtered ADF images of WSe 2 of ( a ) SV Se (white polygon) and DV Se (yellow polygon), ( b ) T 1 defect and ( c ) T 2 defect. ( d – f ) The atomic model of T 0 to T 1 transformation including the creation of three DV Se (red crosses) ( d ) and a 60° rotation of three pairs of W–Se bonds around the W atom (green) e to form T 1 with three octagons (blue; f ). ( g – i ) The atomic model of T 1 to T 2 transformation. ( g ) Two DV Se are created at the vicinity of T 1 defect. ( h ) Seven pairs of W–Se bond rotations according to the W atoms marked by green color. ( i ) The T 2 defect. Scale bar, 0.5 nm. Full size image The trefoil defects persist when the samples are cooled to room temperature ( Supplementary Fig. 3 and Supplementary Note 2 ). We also found that trefoil defects can be produced directly at room temperature. However, in the latter case, the defects usually appear in asymmetric shapes with only two octagon leaves as shown in Supplementary Figs 4,5 and 7 , because the energy barriers for bond rotations are relatively high, and the multistep transformations may require longer times than at high temperatures. To rationalize the experimental findings, we carried out first-principles calculations of the atomic structures and formation energies of the defect structures. We define the formation energy E f of a defect in a TMD MX 2 as where E conf is the energy of the supercell with the defect, E 0 is the energy of the pristine supercell, N X are the number of missing chalcogen atoms and μ X their chemical potential with respect to X 2 molecule. Our calculations show that rotating three W–Se bonds by 60° after 3DV Se were created ( Fig. 2e ) lowers the energy of the system by 1.8 eV. Supplementary Table 1 lists the formation energies of the trefoil and various rotational defects in the S/Se-deficient MoS 2 , MoSe 2 , WS 2 and WSe 2 lattice, for convenience given as normalized per chalcogen vacancy. The T 1 (3DV) has lower formation energy per S/Se vacancy than SV or other defect structures and in particular the T 1 (3SV) defect is strongly unfavourable. For the MoS 2 , the staggered DV line structure [18] shows lower energy than the T 1 (3DV) defect, which may explain that T 1 (MoS 2 ) defect has not been found in our experiments. Expansion of trefoil defects by multiple M–X bond rotations Figure 2c shows a larger second-order rotational defect (T 2 ) in WSe 2 . The T 2 defect has a triangular shape and is about twice the size of T 1 with each edge containing two octagons (six octagons in total, purple) as shown in the model in Fig. 2i . A model of the atomic rearrangement during the transformation from T 1 to T 2 is presented in Fig. 2g–i . When two more DV Se are created near the T 1 (red crosses in Fig. 2g ), the structure can be transformed into T 2 by rotating seven pairs of W–Se bond ( Fig. 2h ) around the three W rotation centres (green atoms in Fig. 2g ). The reverse transformation that restores, for example, T 1 /T 2 to T 0 by another set of M–X bond rotations was also observed (see Supplementary Movie 1 ). When the rotational defect transforms to a larger defect (for example, T 2 to T 3 ), a larger number of collective M–X bond rotations might require higher energy barriers, as a result, the transformation process is divided into more steps of M–X bond rotation (see Supplementary Figs 8 and 9 , Supplementary Movie 2 and Supplementary Note 3 ). Migration of trefoil defects During our STEM observations, not only the Se vacancies but also the trefoil defects were mobile ( Supplementary Figs 6 and 10 , Supplementary Movies 3 and 4 and Supplementary Note 4 ). The migration rate of the trefoil defects is much lower than that of SV or DV, presumably due to the collective rearrangement of a larger number of atoms. 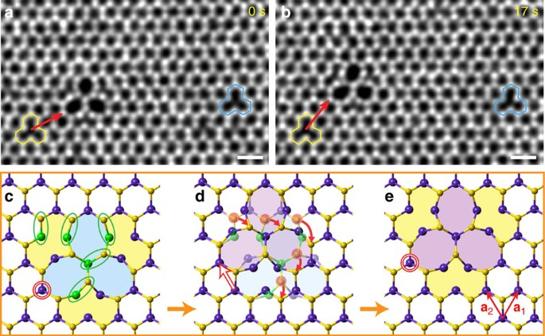Figure 3: Migration of trefoil defect in TMDs. (a,b) T1defect migration in WSe2. The sequential STEM images were carefully aligned according to the vicinal large cluster (not shown) using the ImageJ software. Two Se divacancies (yellow and blue polygons) are stable in the consecutive frames, and used as references. (c–e) The migration model of T1defect glides a lattice constant distance towards the a1direction. Scale bar, 0.5 nm. Figure 3a,b shows an example of in-plane gliding of T 1 (WSe 2 ) by one lattice constant distance (see Supplementary Movie 5 ). Two Se divacancies, highlighted by yellow and blue polygons, were stable in the consecutive ADF images and acted as the reference. The initial and final locations of the trefoil defect are indicated by the red arrows that point to the corners of the octagons according to the yellow divacancy. Figure 3c–e shows an atomic model of T 1 defect gliding. Five pairs of W–S bonds (marked by green circles in Fig. 3c ) rotate collectively clockwise (red arrows in Fig. 3d ) around five W rotation centres (green atoms) to accomplish the migration of the T 1 defect in a distance equal to one lattice constant in the a 2 direction (red hollow arrow). Larger T 2 (WSe 2 ) defects can also migrate in the host lattice ( Supplementary Fig. 11 , and Supplementary Movie 6 ) by a similar mechanism, with multiple M–X bond rotations. Figure 3: Migration of trefoil defect in TMDs. ( a , b ) T 1 defect migration in WSe2. The sequential STEM images were carefully aligned according to the vicinal large cluster (not shown) using the ImageJ software. Two Se divacancies (yellow and blue polygons) are stable in the consecutive frames, and used as references. ( c – e ) The migration model of T 1 defect glides a lattice constant distance towards the a 1 direction. Scale bar, 0.5 nm. Full size image p-type doping and magnetism of large trefoil defect and 8–5–5–8 domain boundary If the M–X bonds rotate further, the rotational defects can expand to even larger sizes. 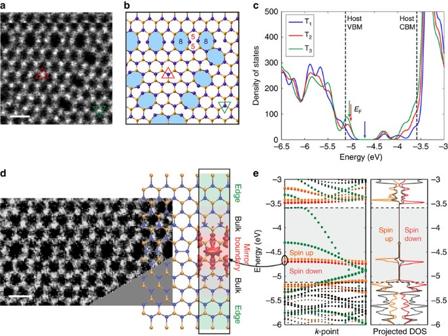Figure 4: Large trefoil defect and magnetic 8–5–5–8 (δ) domain boundary. (a) The ADF image of T4(WSe2). (b) The corresponding atomic model of T4(WSe2) shown ina. Larger rotational defect keep the triangular shape and include three boundaries consisting of 8–5–5–8 membered rings (δ boundary). The orientation of the inner domain of the T4 defect is 60° (or 180°) rotated from the outer domain. (c) Calculated density of states from T1to T3defects. The Fermi-level positions are denoted with arrows. (d) The ADF image of the boundary from T6(WSe2) with the atomic structure partially overlaid. (e) The edge band structure and density of states of the δ boundary with colours denoting projections to different regions within the ribbon geometry used in the calculation. Dashed lines denote the band edge positions of pristine WSe2. The wavefunction isosurface for the mid-gap state localized to the δ boundary is also shown inb. Energy zero is at the vacuum. Scale bar, 0.5 nm. Figure 4a shows an ADF image of T 4 (WSe 2 ) defect. According to the structural parameters for rotational defects listed in Table 1 , the T 4 defect involves 36 pairs of M–X bond rotation around 16 W rotation centres, which leads to a large triangular shape and each edge contains four octagons sandwiched with a pair of pentagons, as illustrated in Fig. 4b . Note that the 8–5–5–8 edges form linear domain boundaries (δ boundary), which are further visualized in Fig. 4d (extracted from the T 6 defect). The calculated density of states from T 1 , T 2 , and T 3 defects in WSe 2 are shown in Fig. 4c . The additional states in the mid gap originate from the corners of the defect, whereas the states close to the valence band maximum and conduction band minimum can be traced to the edges (see Supplementary Figs 12 and 13 ). Interestingly, as the size of the defect increases, the Fermi-level moves closer to the valence band maximum, that is, the edge states of middle-sized defects essentially lead to p-type doping of the system. On the other hand, recent tight-binding transport calculations showed that the conductivity of MoS 2 sheets with large rotational defects and grain boundaries containing 8–5–5–8 rings is strongly reduced across such defects [21] . We did not observe any rotational defects in MoS 2 , but their effects on the electronic transport in other TMDs we studied may be similar. Figure 4: Large trefoil defect and magnetic 8–5–5–8 (δ) domain boundary. ( a ) The ADF image of T 4 (WSe 2 ). ( b ) The corresponding atomic model of T 4 (WSe 2 ) shown in a . Larger rotational defect keep the triangular shape and include three boundaries consisting of 8–5–5–8 membered rings (δ boundary). The orientation of the inner domain of the T4 defect is 60° (or 180°) rotated from the outer domain. ( c ) Calculated density of states from T 1 to T 3 defects. The Fermi-level positions are denoted with arrows. ( d ) The ADF image of the boundary from T 6 (WSe 2 ) with the atomic structure partially overlaid. ( e ) The edge band structure and density of states of the δ boundary with colours denoting projections to different regions within the ribbon geometry used in the calculation. Dashed lines denote the band edge positions of pristine WSe 2 . The wavefunction isosurface for the mid-gap state localized to the δ boundary is also shown in b . Energy zero is at the vacuum. Scale bar, 0.5 nm. Full size image Table 1 Structural parameters for trefoil-like defects. Full size table Figure 4e shows the electronic structure and the local density of states of the ideal δ boundary in WSe 2 . The electronic states localized to the boundary have now energies in the lower mid-gap region with very small dispersion and consequently large density of states. The conductivity along these boundaries will then strongly depend on the Fermi-level position within the gap. These states were also found to carry a magnetic moment. A similar behaviour was reported for the 5–7 dislocation [22] and 8–5–5–8 boundary in MoS 2 (ref. 23 ) and epitaxial graphene on Ni(111) [24] . Calculating the elastic properties of pristine and defective WSe 2 , we found that a Se vacancy concentration of 3%, in the range of the experimentally observed concentrations, decreases the bulk modulus by only about 4%. This indicates that inducing these defect structures only weakly deteriorates the mechanical properties of the system while giving rise to substantial changes in the electronic structure. As shown in the present study by direct visualization of atomic-scale transformations, TMDs feature a rich variety of rotational defects, with the structures and their formation mechanisms related to the symmetry of the lattice but clearly distinct from those in other 2D materials such as graphene and h-BN. Phase transitions [25] and inverse domains may be induced a posteriori, for example, by electron-beam irradiation, which leads to drastic changes in the material properties, for example, p-type doping and magnetism. The bond rotation mechanism reported here not only gives rise to a new class of defects, but also adds to the toolbox of available means for modifying the local properties of TMDs. Material synthesis and sample preparation Single crystal of MoS 2 , MoSe 2 , WS 2 and WSe 2 were grown by chemical vapour transport method using either Br 2 as a transport agent at 950 °C. Ten grams of 99.99% purity of Mo or W, and S or Se elements with 5 mg cm −3 of Br 2 were cooled in a quartz tube ampoule with liquid nitrogen and sealed in vacuum (~1 × 10 −6 Torr) [26] , [27] . Single-layer TMDs were mechanically exfoliated from synthesized crystals using Scotch tape and transferred to 300 nm SiO 2 /Si substrate. To grow WSe 2 by chemical vapour deposition, WO 3 and Se powders were, respectively, used as the tungsten and selenium sources, which were placed in two separate quartz boats located in upstream of a gas flow. The temperatures of the WO 3 and Se powders were set at 850 and 250 °C, respectively. The sapphire substrates where the WSe 2 flakes were deposited at 750 °C were placed at the downstream side with WO 3 and Se vapours being transported by an Ar/H 2 flowing gas (Ar=60 s.c.c.m. and H 2 =3 s.c.c.m.). During the growth, the pressure of reaction chamber keeps constantly at 70 Torr. The specimens were transferred to TEM microgrid and heated in the TEM chamber (vacuum level of ~1.8 × 10 −5 Pa) at 500 °C in a JEOL heating holder. STEM-ADF-imaging experiments STEM-ADF imaging was performed using an aberration-corrected JEOL-2100 F equipped with a DELTA corrector and cold field-emission gun. The microscope was operated at an accelerating voltage of 60 kV. The convergence semi-angle was set to 35 mrad, and the inner acquisition semi-angle was 79 mrad. The probe current was 10–15 pA. The sequential ADF images were recorded with 512 × 512 pixels and acquired with 16–64 μs dwell time. The ADF images in Figs 1 , 2 , 3 have been processed by low-pass filter to enhance the contrast. False-colour images and the image alignment were processed using ImageJ. Computational details Density functional theory calculations were carried out with the PAW method as implemented in the VASP software package [28] , [29] , using the PBE exchange-correlation functional [30] . The defects were modelled in periodically repeated 10 × 10 supercells of the primitive trigonal lattice with the sheets separated by 16 Å of vacuum. A single k-point was used for BZ integration and the plane-wave basis set cutoff was 300 eV. For a few selected structures, the supercell size was increased to 14 × 14 and the energy cutoff increased to 400 eV, which produced an error of at most 0.1 eV, which is our estimated numerical accuracy. Calculations for ideal boundaries were carried out in the ribbon geometry with five MX 2 units on each side of the boundary and with fully chalcogen passivated edge structures, as shown in Fig. 4d . Twelve k-points along the ribbon were found to yield converged results. Robustness of the magnetization was checked by performing additional calculations with 24 k-points and of varying the smearing parameter. The results for MoSe 2 look very similar to the WSe 2 results. How to cite this article : Lin, Y-C. et al . Three-fold rotational defects in two-dimensional transition metal dichalcogenides. Nat. Commun. 6:6736 doi: 10.1038/ncomms7736 (2015).